Cobalt-catalyzed deoxygenative triborylation of allylic ethers to access 1,1,3-triborylalkanes Polyborylated organic compounds have been emerging as versatile building blocks in chemical synthesis. Here we report a selective cobalt-catalyzed deoxygenative 1,1,3-triborylation reaction of allylic ethers with pinacolborane to prepare 1,1,3-triborylalkane compounds. With naturally abundant and/or synthetic cinnamic methyl ethers as starting materials, we have achieved the synthesis of a variety of 1,1,3-triborylalkanes (25 examples). The synthetic utility of these 1,1,3-triborylalkanes is demonstrated through site-selective allylation, protodeborylation, and consecutive carbon-carbon bond-forming reactions. Mechanistic studies including deuterium-labeling and control experiments suggest that this 1,1,3-triborylation reaction proceeds through initial cobalt-catalyzed deoxygenative borylation of allylic ethers to form allylic boronates followed by cobalt-catalyzed 1,1-diborylation of the resulting allylic boronates. Organoboron compounds are important reactive intermediates in chemical synthesis because of their high stability, low toxicity, and versatile reactivity in numerous carbon–carbon or carbon–heteroatom bond-forming reactions [1] . Compared with monoboronate compounds that are widely employed in Suzuki-Miyaura cross-coupling reactions [2] , the synthesis and synthetic potential of polyboron compounds have remained much less explored. gem -Diborylalkanes have recently been emerging as useful reagents for various C–C bond-forming reactions, which in turn has stimulated various methods for their synthesis [3] , [4] , [5] . As another important family of polyboron compounds, triborylalkanes have yet to receive equal attention in organic synthesis principally because straightforward synthetic approaches to prepare them are limited. For example, 1,1,1-triborylalkanes, prepared by the borylation of activated C–H bonds [6] including the benzylic [7] , [8] and homobenzylic [9] C–H bonds or the borylation/hydroboration of alkenes [10] , [11] , [12] and alkynes [13] , [14] , can form stabilized gem -diboryl carbanions through base-induced deborylation under milder basic conditions (Fig. 1a ) [8] . These 1,1,1-triborylalkanes can undergo deborylative Boron–Wittig olefination, alkylation, and conjugated addition reactions [8] , [11] , [15] . 1,1,2-Triborylalkanes, typically synthesized by multi-borylation of alkenes [16] , [17] , alkynes [18] and carbonyl groups [19] , can generate α-boryl carbanions stabilized by five-membered internal chelation through base-induced deborylation of an adjacent boryl group in the gem -diborylalkane unit (Fig. 1a ) [20] , and can subsequently undergo diastereoselective alkylation reactions [16] . In this regard, we consider that 1,1,3-triborylalkanes can also generate α-boryl carbanions stabilized by six-membered internal chelation (Fig. 1a ) and can have similar or even greater synthetic potential as they may undergo sequential C–C bond-forming reactions to allow the installation of three new C–C bonds. However, general approaches to synthesize such 1,1,3-triborylalkanes are lacking and their synthetic utility has remained to be explored. Fig. 1: Introduction and the proposed synthesis of triborylalkane compounds. a Triborylalkane compounds. b Current strategies of relay functionalization and gem -diborylation. c Conceptual design of cobalt-catalyzed deoxygenative 1,1,3-triborylation. Full size image β - X ( X = heteroatoms) elimination from alkylmetal species is involved in numerous transition metal-catalyzed organic transformations [21] , [22] , [23] , [24] , [25] , [26] , [27] and this classic elementary reaction of organometallic species can produce functionalized alkenes (Fig. 1b ), which may undergo further transformations in a tandem manner [17] , [28] , [29] , [30] , [31] . For example, copper-catalyzed allylic borylation of allylic electrophiles is a well-developed method to prepare allylic boronates and mechanistic studies suggest that these allylic borylation reactions proceed with copper-boron intermediates as boron nucleophiles [32] . However, boryl-containing alkenes generated in these allylic borylation reactions do not undergo further borylation to form polyboron compounds under the conditions identified for copper-catalyzed allylic borylation reactions. Recently, catalytic 1,1-diborylation of alkenes has been developed into a straightforward approach to access synthetically versatile gem -diborylalkanes with nickel, cobalt, or zirconium catalysts [33] , [34] , [35] , [36] . These metal-catalyzed 1,1-diborylation reactions occurs through metal-boryl intermediates and migratory insertion of alkenes into such metal-boryl species is the key step to achieve this diborylation transformation. To develop a general approach to access 1,1,3-triborylalkane compounds, we envisioned that metal-catalyzed 1,1-diborylation of branched allylic boronates that are generated in situ via catalytic allylic borylation of allylic electrophiles could afford 1,1,3-triborylalkane products, provided that one transition metal compound can effectively catalyze both 1,1-diborylation and allylic borylation reactions under identical reaction conditions. Allylic alcohol derivatives, such as allyl carbonates, acetates, and phosphates, have been extensively employed as electrophiles for catalytic carbon–carbon and carbon–heteroatom bond-forming reactions [37] . Compared with these commonly used allylic substrates, allyl ethers are considered less reactive and have been explored much less for catalytic organic reactions whereas they are readily accessible, cheap, and easy to handle. Recently, we have reported cobalt-catalyzed 1,1-diborylation of terminal alkenes in the presence of a hydrogen acceptor, and mechanistic studies suggest the competence of a Co-Bpin intermediate [33] . Conceptually, applying this cobalt-boron chemistry to functionalize allylic ethers, which can be derived from naturally abundant cinnamic acid and aldehyde compounds, here we developed a cobalt-catalyzed deoxygenative triborylation reaction of allylic ethers to prepare 1,1,3-triborylalkanes (Fig. 1c ). Migratory insertion of allylic ether into a Co-Bpin species forms an alkylcobalt species containing a β -alkoxy group, and this alkylcobalt species can undergo facile β -alkoxy elimination to produce a branched allyl boronate due to the relatively high oxophilicity of cobalt [38] , [39] . Subsequent 1,1-diborylation of the resulting allyl boronate in the presence of the same cobalt catalyst can afford the desired 1,1,3-triborylalkane product. Evaluation of reaction conditions To initiate the study on this cobalt-catalyzed deoxygenative triborylation reaction, we chose the reaction of allylic compounds ( 2a – 5 ), derived from naturally abundant cinnamyl alcohol ( 1 ), with pinacolborane (HBpin) to identify reaction conditions that favor the formation of 1,1,3-triborylalkane product. The cobalt catalyst employed in this study was generated from bench-stable Co(acac) 3 and xantphos and activated in situ by the reaction with HBpin. These experiments were conducted with allylic substrates as limiting reagents with six equivalents of HBpin in the presence of 5 mol% cobalt catalyst and five equivalents of norbonene (nbe) as a hydrogen acceptor in cyclohexane at 100 °C. 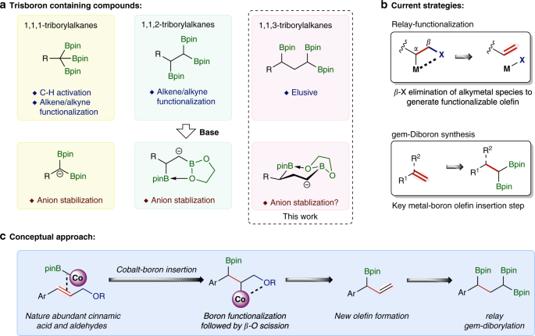Fig. 1: Introduction and the proposed synthesis of triborylalkane compounds. aTriborylalkane compounds.bCurrent strategies of relay functionalization andgem-diborylation.cConceptual design of cobalt-catalyzed deoxygenative 1,1,3-triborylation. The results of selected examples of these experiments are summarized in Table 1 . In general, this reaction produces several organoboron compounds, such as monoborylalkane 6 , 1,3-diborylalkane 7a , 1,1-diborylalkane 7b , 1,1,3-triborylalkane 8a , and 1,1,2-triborylalkane 8a ′. Table 1 Evaluation of conditions for the cobalt-catalyzed triborylation a . Full size table Cinnamyl alcohol 1 reacted to afford a mixture of diborylalkanes ( 7a and 7b ) and 1,1,3-triborylalkane ( 8a ) as a major product (entry 1 in Table 1 ). Subsequently, we tested several cinnamyl alcohol derivatives ( 2a – 5 ) containing various leaving groups for this deoxygenative triborylation reaction (entries 2–5 in Table 1 ). The reaction conducted with cinnamyl methyl ether 2a occurred to full conversion and the desired product 1,1,3-triborylalkane ( 8a ) was formed in 70% GC yield (entry 2 in Table 1 ). Benzoate 3 and phosphate 4 of cinnamyl alcohol did not react with HBpin under identified conditions (entries 3 and 4 in Table 1 ). Silyl ether 5 of cinnamyl alcohol also reacted to give 1,1,3-triborylalkane 8a as the major product (entry 5 in Table 1 ). We also tested various temperatures for the reaction of methyl ether 2a (entries 2 and 6 – 8 in Table 1 ) and found that the reaction at 100 °C produced 8a with a high selectivity. In addition, we found that concentrations of 2a also had noticeable influence on the selectivity of this deoxygenative triborylation and reactions run with more concentrated (0.1 M or 1.0 M) solutions of 2a yielded the target product 8a in lower yields (entries 9 and 10 in Table 1 ). Furthermore, this cobalt-catalyzed deoxygenative triborylation of cinnamyl methyl ether 2a did not occur in the absence of norbornene, and the reaction afforded monoborylalkane 6 as a major product with a high selectivity (>85%), together with trace amounts (<5%) of triborylalkane products (entry 11 in Table 1 ). Monoborylalkane 6 did not undergo further reactions with HBpin to yield 1,1,3-triborylalkane 8a in the presence of norbornene and the cobalt catalyst. Diminished selectivity and yields of 8a were obtained when the reactions were conducted with fewer equivalents of norbornene (entry 12 in Table 1 ) or with fewer equivalents of HBpin (entries 13 and 14 in Table 1 ). With the identified conditions (entry 2 in Table 1 ) for the synthesis of 1,1,3-triborylalkanes, we explored the scope of cinnamic methyl ethers for this cobalt-catalyzed deoxygenative triborylation, and the results are shown in Fig. 2 . In general, a variety of aryl-substituted ( E )-allyl or ( E , Z )-allyl methyl ethers reacted with HBpin in the presence of norbornene to afford the corresponding 1,1,3-triborylalkanes ( 8a – 8u ) in moderate to good isolated yield and high regioselectivity, and the stereochemistry of allyl ether starting materials is inconsequential to the outcome of these reactions. The structure of triborylalkane 8g was confirmed by single crystal X-ray analysis. 1,1,3-Triborylalkane products could be purified by column chromatography on silica, however, their instability on silica columns significantly lowered their isolated yields. Fig. 2: Substrate scope of allylic ethers for this cobalt-catalyzed triborylation reaction. Conditions: a Co(acac) 3 (15.0 μmol), xantphos (15.0 μmol), allylic methyl ether (0.300 mmol), HBpin (1.80 mmol), nbe (1.50 mmol), cyclohexane (10 mL), 100 °C, 2 h, isolated yields, regioselectivity ( 8 : 8 ′) in parentheses; b Solvent cyclohexane/THF (1 : 1). Full size image The data in Fig. 2 showed that both the steric and electronic properties of the aryl substituents in allyl ethers had significant influence on the isolated yields of 1,1,3-triborylalkane products. For example, steric bulkiness at the para -position of aryl groups ( 8a – 8c ) did not have a noticeable influence on the isolated yields, but increasing the steric hindrance at the ortho -position of aryl groups ( 8n and 8o ) decreased the isolated yields. In addition, the substrates containing electron-rich aryl groups ( 8r – 8u ) reacted to provide the desired products in higher isolated yields than the substrates containing electron-deficient aryl groups ( 8i and 8l ). More interestingly, allyl ethers derived from pulp waste lignin components, p- coumaryl ( 8r ), coniferyl ( 8s and 8t ), and sinapyl ( 8u ) monolignols also underwent this cobalt-catalyzed deoxygenative triborylation to produce the corresponding 1,1,3-triborylalkanes in good isolated yields. Aliphatic allylic methyl ethers reacted under identified conditions to give a complex mixture of mono-, di-, and triborylalkane products with the corresponding regioisomers. In addition, allyl methyl ethers with aryl substituents on the 2-position also underwent this cobalt-catalyzed reaction to afford desired 1,1,3-triborylalkane products ( 8v – 8y) , albeit in modest isolated yields. Synthetic utility To highlight the reliability of this deoxygenative triborylation, we tested this protocol with complex substrate 9 , a cholesterol derived allylic ether, and this reaction provided the desired 1,1,3-triborylalkane 10 in a modest yield (Fig. 3a ). We also showed that triborylalkane 8a underwent several further transformations. For example, allylation of 8a with 3-bromo-2-methyl-prop-1-ene in the presence of a non-nucleophilic base LiTMP (TMP = tetramethylpiperidide) to afford a new 1,1,3-triborylalkane 11 in good isolated yield [40] , and compound 11 could undergo stepwise protodeborylation reactions to yield diborylalkane 12 and monoborylalkane 13 in synthetically useful yields (Fig. 3b ). In addition, we also demonstrated that three new C–C bonds could be sequentially constructed by selective conversion of three C–B bonds of 1,1,3-triborylalkanes. For example, allylation of 8a with 3-bromo-2-methyl-prop-1-ene followed by protodeborylation in the presence of NaO t Bu as a base and MeOH as a proton source afforded 1,3-diborylalkane 14 in 55% isolated yield (Fig. 3c ). The relative stereochemistry of 14 was assigned anti by oxidizing 14 to a 1,3-diol and comparing the stereochemistry of the 1,3-diol with the reported data (see Supplementary Fig. 7 for a plausible explanation of this obtained diastereoselectivity) [41] . The benzylic boronate in 14 selectively underwent palladium-catalyzed cross-coupling with 4-iodoanisole to afford alkylboronate 15 , which could further react with 2-thienyllithium to produce compound 16 in high isolated yield (Fig. 3c ) [42] . Fig. 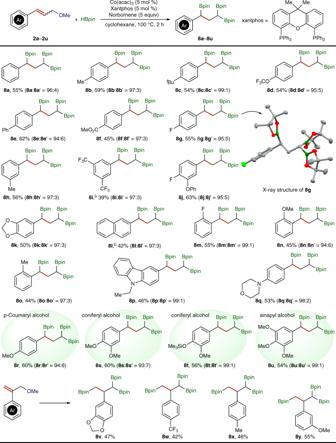Fig. 2: Substrate scope of allylic ethers for this cobalt-catalyzed triborylation reaction. Conditions:aCo(acac)3(15.0 μmol), xantphos (15.0 μmol), allylic methyl ether (0.300 mmol), HBpin (1.80 mmol), nbe (1.50 mmol), cyclohexane (10 mL), 100 °C, 2 h, isolated yields, regioselectivity (8:8′) in parentheses;bSolvent cyclohexane/THF (1 : 1). 3: Synthetic applications of the deoxygenative triborylation method. 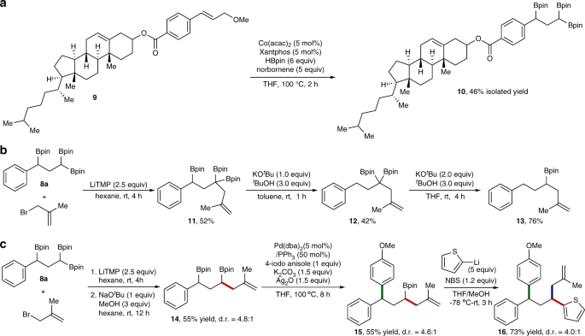Fig. 3: Synthetic applications of the deoxygenative triborylation method. aTriborylation of a cholesterol derived allylic ether.bAllylation of8aand sequential deborylation reactions.cStepwise functionalization of 1,1,3-triborylalkane8awith sequential three new carbon-carbon bond-forming reactions. a Triborylation of a cholesterol derived allylic ether. b Allylation of 8a and sequential deborylation reactions. c Stepwise functionalization of 1,1,3-triborylalkane 8a with sequential three new carbon-carbon bond-forming reactions. Full size image Mechanistic considerations First, we conducted deuterium-labeling studies to get some preliminary understanding of this cobalt-catalyzed deoxygenative triborylation. To find out whether this transformation proceeds through β- O elimination pathway or allylic substitution via π -allyl metal species, we tested this deoxygenative triborylation reaction with 2a - D under standard conditions (Fig. 4a ). One would expect a scrambling of deuterium across the allyl carbons in presences of π -allyl metal intermediates [43] , [44] . The absence of deuterium on the benzylic carbon in 8a - D suggests that the reaction proceed through a β- O elimination pathway instead of an allylic substitution pathway. We also conducted 1,1,3-triborylation of 1a with DBpin in the presence of norbornene under standard conditions, and found that deuterium atoms were incorporated onto all three non-aromatic carbons in substrate 2a (Fig. 4b ). This observed deuterium incorporation can be explained by reversible insertion β- H elimination via a Co-H intermediate. In addition, gas chromatography-mass spectrometry analysis on the crude reaction mixture also revealed the incorporation of deuterium into norbornane molecules. Fig. 4: Mechanistic studies. a The reaction of 2a-D with HBpin. b The reaction of 1a with DBpin. c The proposed catalytic pathways for this cobalt-catalyzed deoxygenative triborylation reaction. Full size image Based on the results of these deuterium-labeling experiments and the precedent of cobalt-catalyzed hydroboration or borylation reactions [7] , [10] , [11] , we proposed plausible catalytic pathways for this cobalt-catalyzed deoxygenative triborylation of allylic ethers. This reaction proceeds through two collaborative catalytic cycles, namely deoxygenative borylation cycle and gem -diborylation cycle (Fig. 4c ). In the deoxygenative borylation cycle, activation of Co(acac) 3 by HBpin in the presence of xantphos generates a cobalt hydride species ( L )Co-H ( I ), which is subsequently converted to a cobalt-boryl species ( L )Co-Bpin ( II ) in the presence of norbornene as a hydrogen acceptor. During this conversion, norbornene is hydrogenated to norbornane. Migratory insertion of cinnamyl methyl ether 2a into ( L )Co-Bpin ( II ) forms an alkylcobalt intermediate ( III ), which undergoes β -OMe elimination to form an allyl boronate 17 and a methoxycobalt species ( L )Co-OMe ( IV ). This methoxycobalt intermediate then reacts with HBpin to regenerate the cobalt hydride ( L )Co-H ( I ) and release a tris(alkoxy)borate MeOBpin ( V ), which can be detected by 11 B NMR spectroscopic analysis with a resonance signal at 22.3 ppm. The gem -diborylation cycle also starts with the conversion of ( L )Co-H ( I ) to ( L )Co-Bpin ( II ) in the presence of norbornene as a hydrogen acceptor. Allyl boronate 17 undergoes migratory insertion into ( L )Co-Bpin ( II ) generates an alkylcobalt species VI , which then isomerizes to a new alkylcobalt species VII via β -H elimination followed by reversible migratory insertion. The alkylcobalt intermediate VII subsequently reacts with HBpin to release 1,1,3-triborylalkane 8a and regenerate the catalytically active ( L )Co-H ( I ). The alkylcobalt species VII contains an α-boryl alkyl group and is thermodynamically stable, which may be caused by the interaction of the d -electrons of Co(I) species with the empty p -orbital on boron. Similar boron-directed isomerization of metal alkyl species was observed previously for other metal-catalyzed chain-walking functionalization of boryl-containing alkenes [45] , [46] , [47] . As shown in Fig. 4c , allyl boronate 17 and vinyl boronate 18 are key intermediates for this cobalt-catalyzed deoxygenative borylation. To support their intermediacy, we then prepared allyl boronate 17 independently and subjected it to the standard reaction conditions, and found that compound 17 was indeed converted to the desired 1,1,3-triborylalkane product with a selectivity of 76% (Fig. 5a ). We also attempted to prepare vinyl boronate 18 , but all the synthetic approaches we have employed did not lead to the formation of compound 18 . 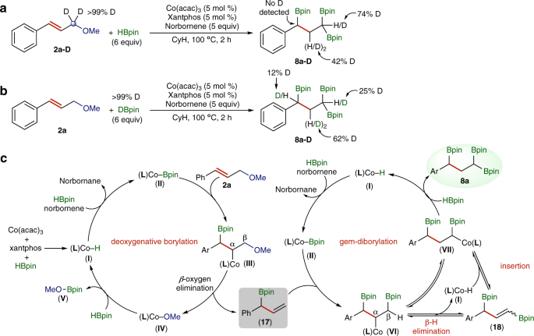Fig. 4: Mechanistic studies. aThe reaction of2a-Dwith HBpin.bThe reaction of1awith DBpin.cThe proposed catalytic pathways for this cobalt-catalyzed deoxygenative triborylation reaction. 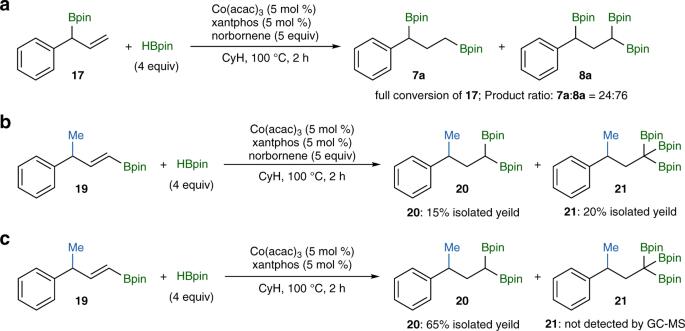Fig. 5: Control experiments to confirm possible reaction intermediates. agem-diborylation reaction of17with HBpin under standard reaction conditions.bThe reaction of19with HBpin in the presence of norbornene as a hydrogen acceptor.cThe reaction of19with HBpin in the absence of norbornene. Alternatively, we synthesized vinyl boronate 19 , which has a structure similar to vinyl boronate 18 , and tested it for this cobalt-catalyzed transformation (Fig. 5b, c ). The reaction of vinyl boronate 19 with excess of HBpin in the presence of norbornene as a hydrogen acceptor yielded gem -diborylalkane 20 and and 1,1,1-triborylalkane 21 with similar isolated yields (Fig. 5b ). However, the corresponding reaction of 19 with HBpin in the absence of norbornene produced only gem -diborylalkane 20 in 65% isolated yield (Fig. 5c ). The results of these two experiments suggest that the isomerization of alkylcobalt species VI to VII , as shown in Fig. 4c , likely proceeds through β -H elimination to form vinyl boronate 18 followed by re-insertion of 18 into cobalt hydride species ( L )Co-H. Fig. 5: Control experiments to confirm possible reaction intermediates. a gem -diborylation reaction of 17 with HBpin under standard reaction conditions. b The reaction of 19 with HBpin in the presence of norbornene as a hydrogen acceptor. c The reaction of 19 with HBpin in the absence of norbornene. Full size image In summary, we have developed an effective protocol for the facile synthesis of 1,1,3-triborylalkanes by cobalt-catalyzed deoxygenative 1,1,3-triborylation of allylic methyl ethers with HBpin. A variety of allylic ethers reacted with HBpin in the presence of norbornene as a hydrogen acceptor to afford synthetically versatile, otherwise challenging to prepare, 1,1,3-triborylalkanes in modest to good isolated yields with high chemo- and regioselectivity. The cobalt catalyst for this deoxygenative triborylation reaction was generated in situ from readily available and bench-stable Co(acac) 3 and xantphos and activated by the reaction with HBpin. Mechanistic studies suggest that this 1,1,3-triborylation reaction proceeds through initial cobalt-catalyzed deoxygenative borylation of allylic ethers to form allyl boronates followed by cobalt-catalyzed gem -diborylation of the resulting allyl boronates. General procedure for dehydrogenative triborylation of allylic ethers In an Argon-filled glovebox, a 20 mL screw-capped vial was charged with Co(acac) 3 (5.3 mg, 15.0 µmol), xantphos (8.7 mg, 15.0 µmol), norbornene (141 mg, 1.50 mmol), allyl methyl ether (0.300 mmol), cyclohexane (10 mL), and a magnetic stirring bar. The solution was stirred and HBpin (261 µL, 1.80 mmol) was added to the vial. The vial was then sealed with a cap containing a PTFE (polytetrafluoroethylene) septum and removed from the glovebox. The mixture was allowed to react at 100 °C for 2 h. Subsequently, the solvent was removed under reduced pressure and the residue was purified by flash chromatography on silica (column I.D. 13.4 mm, eluent:  hexane/ethyl acetate) to afford the corresponding 1,1,3-triborylalkane products. See the Supplementary Information for detailed experimental procedures and the characterization data of all the products.